TGFβ induces the formation of tumour-initiating cells in claudinlowbreast cancer The role of transforming growth factor-beta (TGFβ) in the progression of different molecular subtypes of breast cancer has not been clarified. Here we show that TGFβ increases breast tumour-initiating cell (BTIC) numbers but only in claudin low breast cancer cell lines by orchestrating a specific gene signature enriched in stem cell processes that predicts worse clinical outcome in breast cancer patients. NEDD9, a member of the Cas family of integrin scaffold proteins, is necessary to mediate these TGFβ-specific effects through a positive feedback loop that integrates TGFβ/Smad and Rho-actin-SRF-dependent signals. In normal human mammary epithelium, TGFβ induces progenitor activity only in the basal/stem cell compartment, where claudin low cancers are presumed to arise. These data show opposing responses to TGFβ in both breast malignant cell subtypes and normal mammary epithelial cell subpopulations and suggest therapeutic strategies for a subset of human breast cancers. Cancer stem cells or tumour-initiating cells (TICs) have been identified in breast cancer and several other solid tumours [1] , [2] , [3] , [4] , [5] . Breast TICs (BTICs), identified by their differential ability to generate tumours upon xenotransplantation into immune-deficient mice, were originally characterized as having the EpCAM + /CD44 + /CD24 −/low phenotype [1] . Human breast cancer is a heterogeneous malignancy with at least five different subtypes (luminal A, luminal B, ERBB2, basal and claudin low ) described [6] , [7] , [8] , [9] . It has been suggested that this heterogeneity results from different breast tumour subtypes originating in cells within distinct compartments of the mammary epithelium [6] , [10] , [11] , [12] . Transforming growth factor-beta (TGFβ) has key roles in a variety of cell types and tissues [13] . TGFβ family members bind to a family of membrane receptor serine-threonine protein kinases that activate members of the Smad family of transcription factors (TFs). In cancer, TGFβ has apparently opposite roles, acting both as a tumour suppressor and as a factor that promotes processes such as invasion, metastasis, immune regulation and host–tumour cell interactions [13] , [14] , [15] . In breast cancer, genetic mouse models provide strong support for a tumour suppressor role of epithelial TGFβ signalling in the early stages of mammary gland tumorigenesis [13] . However, both activation and complete depletion of TGFβ signalling enhanced metastasis in mouse models [16] , [17] , [18] . These apparently conflicting reports reveal an incomplete understanding of the role of the TGFβ pathway in breast cancer. A key role of the TGFβ pathway in regulating both normal and cancer stem cell behaviour in different tissues has recently been described [19] , [20] , [21] . Specifically, a role for the TGFβ pathway in the maintenance of BTICs has been suggested, since EpCAM + /CD44 + /CD24 −/low cell subpopulations have an active TGFβ signalling pathway [22] , [23] . However, others have demonstrated that TGFβ suppresses tumorigenesis through inhibition of BTICs in a ER-negative (ER − ) breast cancer model [24] . In the experiments described here, we aimed to reconcile these observations by taking into account breast cancer heterogeneity. We have examined TGFβ effects on BTICs and demonstrate TGFβ has opposing effects on different types of breast cancer. Mechanistically we show that TGFβ/Smad signalling converges with active SRF to increase BTIC numbers in claudin low cell lines through the regulation of a specific gene expression program (TβSC-A). Induction of NEDD9 is necessary to establish a positive feedback loop that links TGFβ/Smad and Rho-actin-SRF signals, which meet at regulatory regions within TβSC-A genes necessary for BTIC activity. Similar opposing effects were observed in normal human mammary epithelial cell subpopulations revealing conserved responses to TGFβ in both malignant and normal mammary epithelial cells. TGFβ differentially regulates mammosphere-initiating cell (MS-IC) numbers To study the effects of TGFβ on stem cell-like traits, we cultured 11 distinct breast cancer cell lines in suspension as floating spheres (mammospheres) as previously described ( Fig. 1a ; Supplementary Table S1 ) [25] . 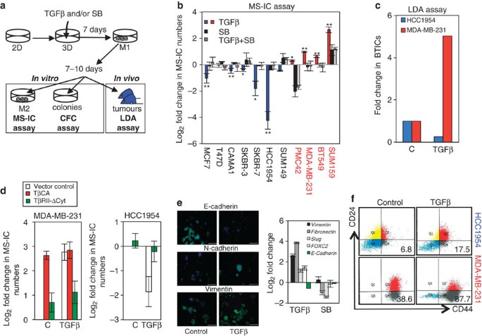Figure 1: Effects of TGFβ pathway activation on human BTICs. (a). Schematic representation of thein vitroandin vivoexperimental approaches that were used in combination to study TGFβ regulation of BTIC behaviour. (b) MS-IC assay. Bar chart shows log2fold changes of M2 mammosphere numbers (which is a read-out of MS-ICs in the M1 cultures) in treated compared with untreated cultures. Error bars represent ±s.d. of at least three independent experiments. **TGFβ-treated versus untreated cultures,P<0.01. *TGFβ-treated versus untreated cultures,P<0.05 (Student'st-test) (c) LDA assay: different doses of single cells from HCC1954 and MDA-MB-231 M1 mammospheres left untreated or treated with TGFβ (2.5 ng ml−1) for 7 days, as indicated, were implanted in the mammary fat pad of NSG mice at limiting dilutions. Bars represent fold change in total number of BTICs in TGFβ-treated M1 as compared with untreated M1 cultures. (d) Same number of single cells from MDA-MB-231- and HCC1945-expressing lenti-HIV-ZsGreen control (vector control), lenti-Tβ1CA (TβCA) or lenti-TβRII-ΔCyt (TβRII-ΔCyt) were grown as M1 mammospheres and left untreated or treated with TGFβ (2.5 ng ml−1) for 7 days as indicated and then processed as in (b). Bar chart shows log2fold changes of MS-ICs in M1 mammospheres compared with vector control untreated M1 cultures. Error bars represent ±s.d. of at least three independent experiments. (e) Immunofluorescence analysis for the expression of E-cadherin, N-cadherin and vimentin in HCC1954 cells grown for 7 days as M1 mammospheres in the absence or presence of TGFβ and then for 24 h in attached conditions. Scale bars, 250 μm (left panel). qRT–PCR assays to assess expression of the indicated transcripts in HCC1954 M1 mammospheres treated with TGFβ (2.5 ng ml−1) or of SB (10 μM) for 4 days. Error bars represent ±s.d. of three independent experiments (right panel). (f) FACS plots of CD44-FITC- and CD24-PE-stained HCC1954 and MDA-MB-231 M1 mammospheres left untreated or treated with TGFβ (2.5 ng ml−1) for 7 days. Numbers indicate the percent of CD44+/CD24−/lowpopulation. Mammosphere cultures were found to be selectively enriched for tumour-initiating cells (TICs) by limiting dilution transplants into the mammary fat pads of NOD/SCID interleukin-2 receptor gamma chain null (Il2rg −/− ) (NSG) mice, when compared with adherent 2D ( Table 1 ). The self-renewal activity and proliferation capacity of cells within the first-generation mammosphere culture (M1) were assayed using MS-IC and colony-forming cell (CFC) assays, respectively [25] , [26] ( Fig. 1a ). We observed that TGFβ decreased the number of both MS-ICs and CFCs in MCF7, CAMA1, SKBR3, SKBR7, HCC1954 and SUM149 cultures. In contrast, TGFβ treatment increased the number of MS-ICs and CFCs in PMC42, MDA-MB-231, BT549 and SUM159 cultures ( Fig. 1b ; Supplementary Fig. S1 ). TGFβ treatment had no effect in T47D cultures. A TGFβ receptor I inhibitor (SB) counteracted TGFβ-mediated changes in MS-IC and CFC numbers ( Fig. 1b and Supplementary Fig. S1 ). Figure 1: Effects of TGFβ pathway activation on human BTICs. ( a ). Schematic representation of the in vitro and in vivo experimental approaches that were used in combination to study TGFβ regulation of BTIC behaviour. ( b ) MS-IC assay. Bar chart shows log 2 fold changes of M2 mammosphere numbers (which is a read-out of MS-ICs in the M1 cultures) in treated compared with untreated cultures. Error bars represent ±s.d. of at least three independent experiments. **TGFβ-treated versus untreated cultures, P <0.01. *TGFβ-treated versus untreated cultures, P <0.05 (Student's t -test) ( c ) LDA assay: different doses of single cells from HCC1954 and MDA-MB-231 M1 mammospheres left untreated or treated with TGFβ (2.5 ng ml −1 ) for 7 days, as indicated, were implanted in the mammary fat pad of NSG mice at limiting dilutions. Bars represent fold change in total number of BTICs in TGFβ-treated M1 as compared with untreated M1 cultures. ( d ) Same number of single cells from MDA-MB-231- and HCC1945-expressing lenti-HIV-ZsGreen control (vector control), lenti-Tβ1CA (TβCA) or lenti-TβRII-ΔCyt (TβRII-ΔCyt) were grown as M1 mammospheres and left untreated or treated with TGFβ (2.5 ng ml −1 ) for 7 days as indicated and then processed as in ( b ). Bar chart shows log 2 fold changes of MS-ICs in M1 mammospheres compared with vector control untreated M1 cultures. Error bars represent ±s.d. of at least three independent experiments. ( e ) Immunofluorescence analysis for the expression of E-cadherin, N-cadherin and vimentin in HCC1954 cells grown for 7 days as M1 mammospheres in the absence or presence of TGFβ and then for 24 h in attached conditions. Scale bars, 250 μm (left panel). qRT–PCR assays to assess expression of the indicated transcripts in HCC1954 M1 mammospheres treated with TGFβ (2.5 ng ml −1 ) or of SB (10 μM) for 4 days. Error bars represent ±s.d. of three independent experiments (right panel). ( f ) FACS plots of CD44-FITC- and CD24-PE-stained HCC1954 and MDA-MB-231 M1 mammospheres left untreated or treated with TGFβ (2.5 ng ml −1 ) for 7 days. Numbers indicate the percent of CD44 + /CD24 −/low population. Full size image Table 1 Frequencies and absolute number of BTICs in mammosphere and adherent 2D cultures. Full size table We observed a correlation between increased self-renewal activity in response to TGFβ with the claudin low signature [9] showing cells with this phenotype respond to TGFβ similarly and in an opposite way compared with other molecular subtypes ( Supplementary Table S1 , Supplementary Fig. S1 and Supplementary Methods ). To investigate the effect of TGFβ on the self-renewal properties of TICs, we transplanted M1 single-cell suspensions from ER − cell lines prototypic of the opposing effects of TGFβ on MS-IC self-renewal (HCC1954-basal and MDA-MB-231-claudin low ) at limiting dilutions into the mammary fat pads of NSG mice ( Fig. 1a ). In HCC1954 M1 cultures, TGFβ mediated a fourfold decrease in the total number of TICs ( Fig. 1c ; Table 1 ). In contrast, in MDA-MB-231 M1 cultures TGFβ induced a fivefold increase in the absolute number of TICs ( Fig. 1c ; Table 1 ). We next modulated the TGFβ pathway in HCC1954 and MDA-MB-231 cells by lentiviral transduction of a constitutive active mutant TGFβ1 (Tβ1CA) or a dominant negative mutant of type II TGFβ receptor (TβRII-ΔCyt) ( Supplementary Methods ) [27] , [28] . TGFβ pathway activation levels were measured by western blotting for p-Smad2 ( Supplementary Fig. S1 ). MDA-MB-231-Tβ1CA showed increased MS-IC and BTIC numbers (compared with MDA-MB-231-vector control) ( Fig. 1d ; Table 1 ). HCC1954-Tβ1CA displayed impaired mammosphere growth precluding propagation for further analysis. The TGFβ effects on MS-IC and BTIC numbers were counteracted by the expression of TβRII-ΔCyt in both cell lines ( Fig. 1d ; Table 1 ). Recently, TGFβ treatment of immortalized human mammary epithelial cells has been shown to induce epithelial-to-mesenchymal transition (EMT) and increase the number of CD44 + /CD24 −/low cells, a phenotype of breast normal and cancer stem cells [1] , [22] . We asked whether the opposing responses to TGFβ in BTIC activity were associated with EMT and/or CD44 + /CD24 −/low phenotypes. TGFβ increased the expression of mesenchymal markers (vimentin, fibronectin, Slug and FOXC2) and decreased the expression of the epithelial marker E-cadherin and increased the number of CD44 + /CD24 −/low cells in the basal cell line HCC1954 ( Fig. 1e,f ). The claudin low cell line, MDA-MB-231, expresses mesenchymal markers and we did not observe significant changes on their expression upon TGFβ treatment, yet in these cells, TGFβ also increased the number of CD44 + /CD24 −/low cells ( Fig. 1f and data not shown). These data show TGFβ-mediated induction of EMT and CD44 + /CD24 −/low phenotypes are separable from its effects on BTICs. TGFβ regulates normal human breast epithelial subpopulations We next asked whether TGFβ would have similar opposing effects in distinct normal breast epithelial cell subpopulations, which are the putative cells of origin of the different breast cancer subtypes. To study the effects of the TGFβ pathway on normal human breast epithelial cell subpopulations, we FACS sorted cells from human reduction mammoplasties using CD49f and EpCAM antibodies ( Fig. 2a ) [29] , [30] . To assess baseline TGFβ pathway activity in these subpopulations we performed qRT–PCR and show that TGFβ downstream targets ( Smad7 , NEDD9 and SERPINA ) were expressed exclusively in the basal compartment (CD49f + /EpCAM neg/low , fraction B in Fig. 2a ), a population that contains myoepithelial cells, myoepithelial-restricted progenitors and mammary stem cells (MaSCs) ( Fig. 2b ). The expression of these transcripts was undetectable in the non-clonogenic ER + luminal cell population (CD49f − /EpCAM + , fraction C) or the luminal progenitor population (CD49f + /EpCAM + , fraction A). Recently, CD49f + /EpCAM neg/low , but not CD49f + /EpCAM + cells, have been shown to express high levels of nuclear Smad2 [21] . Together with our data, this confirms the presence of an active TGFβ pathway in the basal but not in the luminal progenitor compartment. We next determined the effects of ectopic activation of the TGFβ pathway in these subpopulations using an in vitro CFC assay. We observed TGFβ treatment decreased the number of colonies generated from the CD49f + /EpCAM + subpopulation and increased the number of colonies generated from the CD49f + /EpCAM neg/low cell subpopulation ( Fig. 2c ). Similar results were obtained from the analogous mouse epithelial cell subpopulations ( Supplementary Fig. S2 ). However, TGFβ decreased total cell numbers in both compartments ( Supplementary Fig. S2 ). We noted the few colonies derived from TGFβ-treated CD49f + /EpCAM + cells were scattered and of mesenchymal appearance, morphologically identical to the colonies generated from the basal compartment ( Fig. 2d [29] ). Consistently, these colonies expressed the basal marker cytokeratin 14 ( Fig. 2e ). 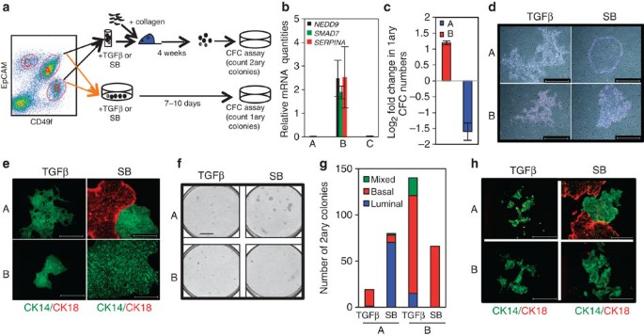Figure 2: TGFβ effects on normal human mammary epithelium. (a) FACS profile of human mammary epithelial cell preparations (depleted of CD45+and CD31+cells) showing the gates used to select normal human mammary epithelial cell subfractions; A: CD49f+/EpCAM+, B: CD49f+/EpCAMneg/lowand C: CD49f−/EpCAM+, and schematic representation of thein vitroandin vivoexperimental approaches that were used to obtain primary and secondary CFCs, respectively. (b) qRT–PCR of the indicated transcripts in epithelial sub fractions as depicted in (a). Expression was normalized against beta-2-microglobulin and displayed as arbitrary units. Error bars represent ±s.d. of three independent experiments. (c) TGFβ (2.5 ng ml−1) was added (at day 0) to flow-sorted subfractions as depicted in (a) and plated at clonogenic densities in the presence of feeder cells (irradiated fibroblasts) in collagen-coated plates for 7–10 days. Colonies were stained with Giemsa and counted. Results are represented as the log2fold changes of primary colonies (or CFCs) in TGFβ-treated compared with untreated cells. Error bars represent ±s.d. of three independent experiments. (d) Microscopy images of Giemsa-stained primary colonies from CFC assays of flow-sorted TGFβ- (2.5 ng ml−1) or SB-(10 μM)-treated cells from fractions A or B. Scale bars, 1 mm. (e) Immunostaining for expression of cytokeratin 14 (green) and cytokeratin 18 (red) of primary colonies from CFC assays of flow-sorted TGFβ- (2.5 ng ml−1) or SB (10 μM)-treated fractions A and B cells. Scale bars, 1 mm. (f) Representative images of secondary colonies of TGFβ- (2.5 ng ml−1) or SB (10 μM)-treated mammary epithelial subpopulation A and B. Scale bars, 1 cm. (g) Bar chart showing number and type (according to their morphology) of secondary colonies of a representative secondary CFC assay of TGFβ- and SB-treated mammary epithelial fractions A and B. (h) Immunofluorescence using antibodies against cytokeratin 14 (CK14) and cytokeratin 18 (CK18) of representative colonies derived from (g). Scale bars, 1 mm Figure 2: TGFβ effects on normal human mammary epithelium. ( a ) FACS profile of human mammary epithelial cell preparations (depleted of CD45 + and CD31 + cells) showing the gates used to select normal human mammary epithelial cell subfractions; A: CD49f + /EpCAM + , B: CD49f + /EpCAM neg/low and C: CD49f − /EpCAM + , and schematic representation of the in vitro and in vivo experimental approaches that were used to obtain primary and secondary CFCs, respectively. ( b ) qRT–PCR of the indicated transcripts in epithelial sub fractions as depicted in ( a ). Expression was normalized against beta-2-microglobulin and displayed as arbitrary units. Error bars represent ±s.d. of three independent experiments. ( c ) TGFβ (2.5 ng ml −1 ) was added (at day 0) to flow-sorted subfractions as depicted in ( a ) and plated at clonogenic densities in the presence of feeder cells (irradiated fibroblasts) in collagen-coated plates for 7–10 days. Colonies were stained with Giemsa and counted. Results are represented as the log 2 fold changes of primary colonies (or CFCs) in TGFβ-treated compared with untreated cells. Error bars represent ±s.d. of three independent experiments. ( d ) Microscopy images of Giemsa-stained primary colonies from CFC assays of flow-sorted TGFβ- (2.5 ng ml −1 ) or SB-(10 μM)-treated cells from fractions A or B. Scale bars, 1 mm. ( e ) Immunostaining for expression of cytokeratin 14 (green) and cytokeratin 18 (red) of primary colonies from CFC assays of flow-sorted TGFβ- (2.5 ng ml −1 ) or SB (10 μM)-treated fractions A and B cells. Scale bars, 1 mm. ( f ) Representative images of secondary colonies of TGFβ- (2.5 ng ml −1 ) or SB (10 μM)-treated mammary epithelial subpopulation A and B. Scale bars, 1 cm. ( g ) Bar chart showing number and type (according to their morphology) of secondary colonies of a representative secondary CFC assay of TGFβ- and SB-treated mammary epithelial fractions A and B. ( h ) Immunofluorescence using antibodies against cytokeratin 14 (CK14) and cytokeratin 18 (CK18) of representative colonies derived from ( g ). Scale bars, 1 mm Full size image To directly investigate TGFβ effects on the number of progenitors and MaSCs, we used a xenotransplantation-based protocol previously described for the quantification of human mammary cells with in vivo regenerative capacity [30] , [31] . Briefly, flow-sorted human breast epithelial cells were exposed to TGFβ or SB for 3 h. Next, the cells were embedded into collagen gels along with supportive fibroblasts, and the gels transplanted under the renal capsule of estrogen- and progesterone-supplemented NSG mice. After 4 weeks, the gels were removed and dissociated, and the liberated cells were seeded into secondary CFC assays (as depicted in Fig. 2a ). TGFβ treatment, in vivo resulted in a decrease in the clonogenic output (CFCs/outgrowth) of CD49f + /EpCAM + and an increase in CD49f + /EpCAM neg/low cells, compared with their SB-treated counterparts ( Fig. 2f,g ). Morphologically [32] , we observed a similar trend in secondary CFCs: colonies derived from TGFβ-treated luminal progenitor outgrowths were exclusively basal, whereas SB-treated outgrowths generated predominantly luminal colonies ( Fig. 2g,h ). Altogether these results show TGFβ differentially regulates human normal mammary epithelial cell subpopulations independently of its cytostatic effects (which are similar in both): it decreases luminal progenitor proliferation and clonogenic capacity and alters their phenotype, and it increases the clonogenic output of MaSC/basal progenitors within the basal compartment. Similar TGFβ signalling in different BTICs We next determined whether the differential effects of TGFβ on BTICs were due to intrinsic differences in the activity of the TGFβ signalling pathway. TGFβ receptors were functional, as shown by increased p-Smad2 levels after TGFβ treatment in all cell lines except T47D. T47D cells do not express TβRII making them unresponsive to TGFβ [33] . Western blotting revealed that total levels of Smads were variable among cell lines, although no significant differences were found between cells with increased and cells with decreased BTIC activity upon TGFβ treatment ( Supplementary Fig. S3 ). To demonstrate whether the TGFβ effects on BTICs are Smad-dependent, we used short interfering RNA (siRNA) to knock down Smad2, Smad3, Smad2 and 3 together and Smad4, and this greatly impaired the effects of TGFβ on M1 on both HCC1954 and MDA-MB-231 cells ( Fig. 3a ; Supplementary Fig. S3 ). Using a reporter assay, we also confirmed that Smads were similarly transcriptionally active in M1 from both TGFβ-treated cell lines ( Fig. 3b ). 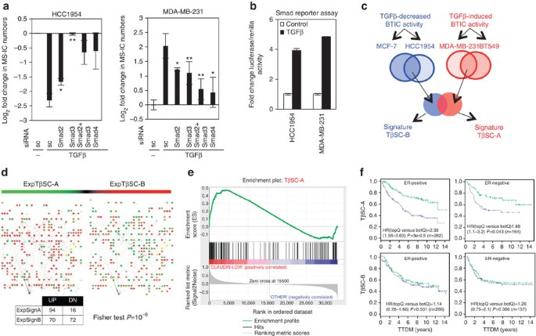Figure 3: TβSC-A is prognostic in breast cancer. (a) Bar chart shows log2fold change of MS-ICs in TGFβ-treated compared with untreated HCC1954 and MDA-MB-231 M1 cultures transfected with the indicated siRNAs. Data represents the mean ±s.d. of three independent experiments. **TGFβ-treated scramble siRNA (sc) cultures versus TGFβ-treated siSmad cultures,P<0.01.*TGFβ-treated scramble siRNA (sc) cultures versus TGFβ-treated siSmad cultures,P<0.05 (Student'st-test). (b) Luciferase activity of untreated (Control) or TGFβ-(2.5 ng ml−1) treated 4-day M1 mammospheres from HCC1954 and MDA-MB-231 transfected (at day 2) with a Smad reporter vector (CAGA12-Luc) normalized to pGL-SV40 renilla transfection control. Results are expressed as fold change from untreated cultures. Data represents the mean ±s.d. of three independent experiments. (c) Schematic representation of the experimental design used to derive TGFβ-specific signatures. Blue- and red-line Venn diagrams represent differentially expressed genes (DEG) in TGFβ- versus SB-treated M1 mammospheres. TβSC-A and TβSC-B signatures were obtained from the list of DEG common and unique to MDA-MB-231 and BT549 (red circle) or common and unique to MCF-7 and HCC1954 (blue circle), respectively. (d) Heat-map-like (red represents upregulated, green represents downregulated) visualization of 'Plurinet' genes for expression data from ExpTβSC-A and ExpTβSC-B. (e) Enrichment plot of upregulated genes from TβSC-A shows a significant enrichment (FDRq-value: 0.05) in the claudinlowsubtype (104 tumours) versus the rest of the Metabric tumours (893)36. The top panel displays the enrichment score. The middle panel shows the position of the genes in the signature in the ranked list of all the genes in the microarray (33,075). The lower panel displays the value of the signal to noise ratio, a measure of the correlation of each gene with the claudinlowsubtype. (f) Kaplan–Meier estimates of time to distant metastasis (TTDM) for top (blue or topQ) and low (green or botQ) quartiles of TβSC-A and TβSC-B activation levels as measured by Spearman rank correlation. Hazard ratio (HR), 95% confidence interval,P-values (Wald test) and numbers of patients are also included. Values of a stratified Cox-regression model where all samples are included, and stratification is done according to cohort are: TβSC-A-ER+: HR=1.319 (1.15–1.5)P=7e-05n=532; TβSC-A-ER−: HR=1.19 (1.01–1.41)P=0.043n=328; TβSC-B-ER+: HR=1.07 (0.93–1.22)P=0.366n=532; TβSC-B-ER−: HR=1.07 (0.93–1.22)P=0.366n=532. Figure 3: TβSC-A is prognostic in breast cancer. ( a ) Bar chart shows log 2 fold change of MS-ICs in TGFβ-treated compared with untreated HCC1954 and MDA-MB-231 M1 cultures transfected with the indicated siRNAs. Data represents the mean ±s.d. of three independent experiments. **TGFβ-treated scramble siRNA (sc) cultures versus TGFβ-treated siSmad cultures, P <0.01. *TGFβ-treated scramble siRNA (sc) cultures versus TGFβ-treated siSmad cultures, P <0.05 (Student's t -test). ( b ) Luciferase activity of untreated (Control) or TGFβ-(2.5 ng ml −1 ) treated 4-day M1 mammospheres from HCC1954 and MDA-MB-231 transfected (at day 2) with a Smad reporter vector (CAGA 12 -Luc) normalized to pGL-SV40 renilla transfection control. Results are expressed as fold change from untreated cultures. Data represents the mean ±s.d. of three independent experiments. ( c ) Schematic representation of the experimental design used to derive TGFβ-specific signatures. Blue- and red-line Venn diagrams represent differentially expressed genes (DEG) in TGFβ- versus SB-treated M1 mammospheres. TβSC-A and TβSC-B signatures were obtained from the list of DEG common and unique to MDA-MB-231 and BT549 (red circle) or common and unique to MCF-7 and HCC1954 (blue circle), respectively. ( d ) Heat-map-like (red represents upregulated, green represents downregulated) visualization of 'Plurinet' genes for expression data from ExpTβSC-A and ExpTβSC-B. ( e ) Enrichment plot of upregulated genes from TβSC-A shows a significant enrichment (FDR q -value: 0.05) in the claudin low subtype (104 tumours) versus the rest of the Metabric tumours (893) [36] . The top panel displays the enrichment score. The middle panel shows the position of the genes in the signature in the ranked list of all the genes in the microarray (33,075). The lower panel displays the value of the signal to noise ratio, a measure of the correlation of each gene with the claudin low subtype. ( f ) Kaplan–Meier estimates of time to distant metastasis (TTDM) for top (blue or topQ) and low (green or botQ) quartiles of TβSC-A and TβSC-B activation levels as measured by Spearman rank correlation. Hazard ratio (HR), 95% confidence interval, P -values (Wald test) and numbers of patients are also included. Values of a stratified Cox-regression model where all samples are included, and stratification is done according to cohort are: TβSC-A-ER+: HR=1.319 (1.15–1.5) P =7e-05 n =532; TβSC-A-ER−: HR=1.19 (1.01–1.41) P =0.043 n =328; TβSC-B-ER+: HR=1.07 (0.93–1.22) P =0.366 n =532; TβSC-B-ER−: HR=1.07 (0.93–1.22) P =0.366 n =532. Full size image We noted that pathway activation was sustained during the M1 culture and persisted 7 days after the single dose of recombinant TGFβ was added to the culture on day 1 ( Supplementary Fig. S3 ), suggesting induction of a positive autocrine TGFβ signalling feedback loop. To test this hypothesis, MDA-MB-231 cells, untreated or treated with recombinant TGFβ bound to biotin (TGFβB) were grown in mammosphere medium and supernatants collected at days 1, 2, 5 and 7. Exogenous TGFβB was removed using magnetic streptavidin-beads, and levels of TGFβ1, 2 and 3 in the supernatant were measured using a multiplex immunoassay. The levels of endogenously secreted TGFβ1 and 2 (TGFβ3 levels were undetectable) increased throughout the 7 days of the experiment ( Supplementary Fig. S3 and Supplementary Methods ). These results suggest that the persistent pathway activation in TGFβ-treated M1 mammospheres is due to a positive feedback loop of autocrine TGFβ signalling. As we observe similar levels of p-Smad2 upon a single dose of TGFβ in M1 derived from cell lines with opposing responses to TGFβ, autocrine activation of TGFβ production and subsequent sustained TGFβ pathway activation in mammosphere cultures is not related to the differential TGFβ effects on BTICs. In summary, these results demonstrate that the opposing effects of TGFβ on BTIC regulation are not explained by differences in the activity of TGFβ receptors, Smad activity or the positive feedback loop of autocrine TGFβ. A TGFβ expression signature for self-renewal of MS-ICs As the differential effects of TGFβ on BTICs from distinct breast cancer cell lines are Smad-dependent, and could not be assigned to differences in Smad transcriptional activity, we hypothesized that the differences could result from distinct TGFβ/Smad-specific transcriptional programs. We profiled, using microarrays, M1 cultures from two cell lines prototypic of TGFβ-mediated decrease (MCF-7 and HCC1954) and two cell lines prototypic of TGFβ-mediated increase (MDA-MB-231 and BT549) in BTIC activity ( Fig. 1b ) (Accession in ArrayExpress E-MTAB-516 and E-MTAB-1190 ). We focused on genes differentially regulated (1% false discovery rate (FDR) and >1 log-fold-change) by TGFβ versus SB. There were 114 TGFβ-specific genes common and unique to MCF-7 and HCC1954 (TGFβ-specific cancer stem cell signature-B or TβSC-B) and 130 TGFβ-specific genes common and unique to MDA-MB-231 and BT549 (TGFβ-specific cancer stem cell signature-A or TβSC-A) ( Fig. 3c ; Supplementary Data 1 ). Gene set enrichment analysis (GSEA) on these signatures using the Molecular Signatures Database [34] showed both TβSC-A and -B signatures are TGFβ-specific signatures ( Supplementary Data 2 ). Moreover, the most significantly enriched gene list in TβSC-A was a signature for stemness (53-gene overlap, P <10 −28 , FDR <0.05), which was only marginally enriched in TβSC-B (13-gene overlap, P <10 −4 , FDR <0.05) ( Supplementary Data 2 ). Analysis using MetaCore data mining technology, which has previously been used in the field [23] , showed one of the most significantly enriched pathways in TβSC-A was EMT in cancer cells ( P <0.0003, FDR <0.05) ( Supplementary Table S2 ; Supplementary Fig. S3 ). To explore these signatures further, we used a recently derived protein–protein interaction subnetwork characterizing pluripotency and stemness (the 'PluriNet') [35] and found it was preferentially upregulated only in TβSC-A ( Fig. 3d ). Interestingly, using our Metabric data set [36] , we observed TβSC-A upregulated genes are enriched in human claudin low tumours (which are the most undifferentiated subtype of breast cancer) compared with the other molecular subtypes ( Fig. 3e ). BTIC numbers have been suggested to vary between breast cancers, and correlate with clinical aggressiveness [37] . We hypothesized that the TβSC-A signature, as linked to increase in BTIC numbers, would correlate with clinical outcome. Kaplan–Meier analysis of tumours with the 25% extreme high and low correlation values with TβSC-A, showed this synexpression signature was associated with time to distant metastasis in both ER − and ER + tumours. In contrast, TβSC-B showed no significant associations ( Fig. 3f ; Supplementary Methods ). We further assessed p-Smad2 expression by immunohistochemistry as a readout of canonical TGFβ pathway activation in 1714 breast cancer cores on TMAs and saw no significant correlation with overall survival in either ER − or ER + breast cancer patients ( Supplementary Fig. S3 and Supplementary Methods ). Thus, canonical TGFβ pathway activation levels (measured by p-Smad2) cannot be used as a prognostic marker in breast cancer, contrasting with synexpression signature TβSC-A, which confers poor prognosis, further strengthening its biological significance. SRF and Smad signalling increase BTIC numbers The TGFβ-specific synexpression signatures represent two distinct cellular context-dependent TGFβ-induced gene responses and are likely to be jointly controlled by a specific Smad-cofactor (TF) combination [13] . To identify these TFs, we used the regulatory network approach ( Fig. 4a ) that compares the differential expression levels of predicted TF targets to the non-targets in TβSC-A and TβSC-B [38] , [39] . This revealed that SRF (serum response factor) targets were the most significantly differentially expressed in TβSC-A ( P <0.01, t -test). Predicted targets of SRF were not differentially expressed in TβSC-B, suggesting that the regulation of SRF targets in response to TGFβ is specific to claudin low cell lines ( Fig. 4a ; Supplementary Fig. S4 and Supplementary Data 3 ). 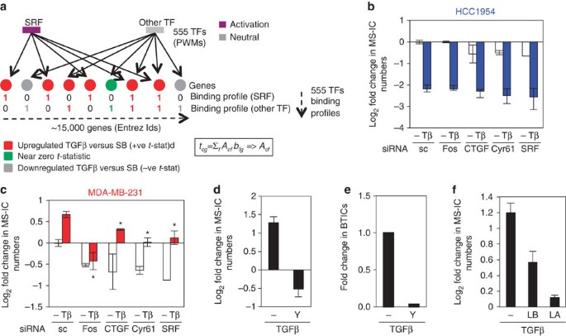Figure 4: MRTF-SRF signalling mediates TGFβ increased in BTIC self-renewal. (a) Regulatory network analysis used to infer differential activity of position weight matrices (PWMs) between two conditions (TGFβ versus SB) in a given cell line (c). The regularizedt-statistics of differential expression of ~15,000 genes between the two conditions (t)is regressed against the binding profiles, (b),of ~555 PWMs (f=1,....,555,coded as 1 s-bound and 0 s-unbound) to infer differential activity of PWMs. Differential activity estimates are provided by the regression coefficients (A). (b) Bar chart shows log2fold change of MS-ICs in M1 cultures of untreated (−) and TGFβ-treated (Tβ) HCC1954 (b) and MDA-MB-231 (c) transfected with siRNAs to knockdownFos, CTGF,Cyr61andSRFas indicated, compared with scramble siRNA (sc)-untreated M1 cultures. Data represents the mean ±s.d. of three independent experiments. *TGFβ-treated scramble siRNA (sc) versus TGFβ-treated siRNA (Fos, CTGF, Cyr61 and SRF),P<0.05 (Student'st-test). (d) Bar chart shows log2fold change of MS-ICs in TGFβ-treated MDA-MB-231 M1 cultures in the presence of 25 μM Y-27632 compared with M1-untreated cultures (−). Error bars represent ±s.d. of three independent experiments. (e) LDA assay using different doses of single cells derived from MDA-MB-231 M1 mammospheres cells left untreated or treated with TGFβ (2.5 ng ml−1) in the absence (−) or presence of Y-27632 for 7 days. Bars represent fold change in total number of BTICs in M1 cultures as compared with M1 untreated cultures. (f) Bar chart shows log2fold change of MS-ICs in TGFβ-treated MDA-MB-231 M1 cultures in the absence (−) or presence of 0.5 μM latrunculin B (LB) or of 0.4 μM latrunculin A (LA) compared with untreated cells. Error bars represent ±s.d. of at least three independent experiments. Figure 4: MRTF-SRF signalling mediates TGFβ increased in BTIC self-renewal. ( a ) Regulatory network analysis used to infer differential activity of position weight matrices (PWMs) between two conditions (TGFβ versus SB) in a given cell line ( c) . The regularized t -statistics of differential expression of ~15,000 genes between the two conditions ( t) is regressed against the binding profiles, ( b), of ~555 PWMs ( f=1,....,555, coded as 1 s-bound and 0 s-unbound) to infer differential activity of PWMs. Differential activity estimates are provided by the regression coefficients ( A ). ( b ) Bar chart shows log 2 fold change of MS-ICs in M1 cultures of untreated (−) and TGFβ-treated (Tβ) HCC1954 ( b ) and MDA-MB-231 ( c ) transfected with siRNAs to knockdown Fos, CTGF , Cyr61 and SRF as indicated, compared with scramble siRNA (sc)-untreated M1 cultures. Data represents the mean ±s.d. of three independent experiments. *TGFβ-treated scramble siRNA (sc) versus TGFβ-treated siRNA (Fos, CTGF, Cyr61 and SRF), P <0.05 (Student's t -test). ( d ) Bar chart shows log 2 fold change of MS-ICs in TGFβ-treated MDA-MB-231 M1 cultures in the presence of 25 μM Y-27632 compared with M1-untreated cultures (−). Error bars represent ±s.d. of three independent experiments. ( e ) LDA assay using different doses of single cells derived from MDA-MB-231 M1 mammospheres cells left untreated or treated with TGFβ (2.5 ng ml −1 ) in the absence (−) or presence of Y-27632 for 7 days. Bars represent fold change in total number of BTICs in M1 cultures as compared with M1 untreated cultures. ( f ) Bar chart shows log 2 fold change of MS-ICs in TGFβ-treated MDA-MB-231 M1 cultures in the absence (−) or presence of 0.5 μM latrunculin B (LB) or of 0.4 μM latrunculin A (LA) compared with untreated cells. Error bars represent ±s.d. of at least three independent experiments. Full size image To investigate this further, we performed MS-IC assays in siSRF-MDA-MB-231 cells and observed a 50% reduction in TGFβ-mediated increase in MS-IC numbers compared with control siRNA-transfected cells. In HCC1954, SRF knockdown did not affect TGFβ-mediated decrease in self-renewal of MS-ICs ( Fig. 4b,c ). We next wanted to investigate whether the SRF-dependent increase in claudin low BTIC activity in response to TGFβ relies on Rho-actin-MRTF (myocardin-related TFs) signals, as SRF activity is controlled by the Rho-actin pathway in MDA-MB-231 cells [40] . We observed TGFβ treatment increased Rho activity in MDA-MB-231 but not in HCC1954 M1 mammospheres ( Supplementary Fig. S4 ). Indeed, siRNAs against Rho-A, Rho-C and Rho-actin-MRTF-SRF downstream targets ( Fos , CTGF and Cyr61) [40] specifically abrogated TGFβ-mediated effects in MS-IC numbers in MDA-MB-231, but not in HCC1954 ( Fig. 4b,c and Supplementary Fig. S4 ). Furthermore, inhibition of the Rho effector ROCK (Rho-kinase) using the inhibitor Y-27632, strongly inhibited the increase in MS-IC and BTIC numbers upon TGFβ treatment ( Fig. 4d,e ; Table 1 ). Treatment with actin-modifier drugs Latrunculin A and B (LA and LB), which inhibit SRF activation through MRTFs, partially blocked TGFβ-mediated increase in MS-IC numbers ( Fig. 4f ). Altogether, these results show Rho-actin-MRTF-SRF signalling is necessary for TGFβ-mediated increase in BTIC activity exclusively in claudin low cells. MRTF-SRF and Smad induce NEDD9 in claudin low cancer cells Our transcriptomic approach showed the gene NEDD9 (neural precursor cell expressed developmentally downregulated 9) to be one of the top ten differentially expressed genes in the claudin low cell lines, but not in others ( Supplementary Data 1 ). This result was validated by qRT–PCR ( Supplementary Fig. S5 ). Significantly, NEDD9 was also overexpressed in claudin low tumours compared with other subtypes of breast cancer ( Supplementary Fig. S5 ). We next confirmed NEDD9 is a Smad and SRF target with a siRNA approach. SRF and Smad downregulation in M1 MDA-MB-231 cells impaired TGFβ-mediated increase in NEDD9 protein and mRNA levels ( Fig. 5a,b ). To assess whether NEDD9 is also an MRTF target, we treated HCC1954 cells with cytochalasin-D (CD) and observed it increased NEDD9 levels ( Fig. 5c ). CTGF and Smad7 were used as controls. MDA-MB-231 cells treated with LB partially blocked TGFβ-mediated increased expression of NEDD9 and several other MRTF-SRF target genes ( Fos , CTGF and Cyr61 ). FOSS gene expression however was not affected ( Fig. 5c ). These results show that MRTF activity is necessary and sufficient to promote an increase in NEDD9 levels. 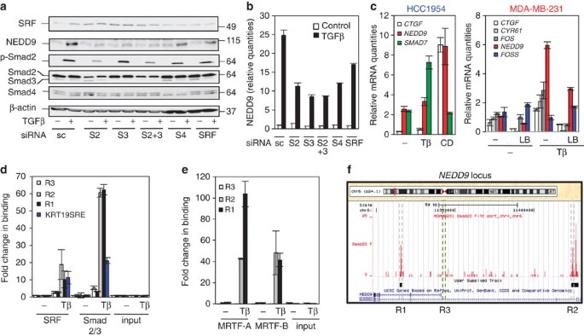Figure 5: NEDD9 is a TGFβ/Smad and MRTF-SRF target. (a) Western blot using the indicated antibodies of untreated (−) and TGFβ (2.5 ng ml−1)-treated (+) MDA-MB-231 M1 cultures transfected with siRNA pools against SRF, Smad2 (S2), Smad3 (S3) Smad2 and 3 (S2+3) and Smad4 (S4). (b) qRT–PCR analysis ofNEDD9in same conditions as in (a). Error bars represent ±s.d. of three experiments. (c) qRT–PCR of the indicated transcripts in HCC1954 (left panel) and MDA-MB-231 (right panel) M1 mammospheres treated with TGFβ (2.5 ng ml−1), 5 μM CD or 0.5 μM LB as indicated. Expression was normalized against beta-2-microglobulin and expressed as arbitrary units. Error bars represent ±s.d. of at least three independent experiments. (d) ChIP assay on MDA-MB-231 M1 mammospheres, untreated (−) or treated with TGFβ (2.5 ng ml−1) (Tβ) for 1 h to detect binding of endogenous SRF and Smad2/3 to R1, R2 and R3. KRT19SBE region was used as an internal positive control for Smad2/3 binding. Results are expressed as TGFβ-induced fold change in binding from untreated control cultures. Error bars represent ±s.d. of three independent experiments. (e) ChIP assay as described in (d) to detect binding of endogenous MRTF-A and MRTF-B. (f) UCSC Genome Browser display showing regions R1, R2 and R3 that were selected to design primers to detect binding of Smad, SRF, MRTF-A and MRTF-B by ChIP-qPCR assays. Error bars represent ±s.d. of three independent experiments. Also showing ChIP-sequencing enrichment of Smad2/3 binding in M1 mammosphere cultures treated with TGFβ (2.5 ng ml−1) for 1 h across theNEDD9genomic region. Black boxes correspond to called binding events obtained using both MACS and SWEMBL algorithms. Figure 5: NEDD9 is a TGFβ/Smad and MRTF-SRF target. ( a ) Western blot using the indicated antibodies of untreated (−) and TGFβ (2.5 ng ml −1 )-treated (+) MDA-MB-231 M1 cultures transfected with siRNA pools against SRF, Smad2 (S2), Smad3 (S3) Smad2 and 3 (S2+3) and Smad4 (S4). ( b ) qRT–PCR analysis of NEDD9 in same conditions as in ( a ). Error bars represent ±s.d. of three experiments. ( c ) qRT–PCR of the indicated transcripts in HCC1954 (left panel) and MDA-MB-231 (right panel) M1 mammospheres treated with TGFβ (2.5 ng ml −1 ), 5 μM CD or 0.5 μM LB as indicated. Expression was normalized against beta-2-microglobulin and expressed as arbitrary units. Error bars represent ±s.d. of at least three independent experiments. ( d ) ChIP assay on MDA-MB-231 M1 mammospheres, untreated (−) or treated with TGFβ (2.5 ng ml −1 ) (Tβ) for 1 h to detect binding of endogenous SRF and Smad2/3 to R1, R2 and R3. KRT19SBE region was used as an internal positive control for Smad2/3 binding. Results are expressed as TGFβ-induced fold change in binding from untreated control cultures. Error bars represent ±s.d. of three independent experiments. ( e ) ChIP assay as described in ( d ) to detect binding of endogenous MRTF-A and MRTF-B. ( f ) UCSC Genome Browser display showing regions R1, R2 and R3 that were selected to design primers to detect binding of Smad, SRF, MRTF-A and MRTF-B by ChIP-qPCR assays. Error bars represent ±s.d. of three independent experiments. Also showing ChIP-sequencing enrichment of Smad2/3 binding in M1 mammosphere cultures treated with TGFβ (2.5 ng ml −1 ) for 1 h across the NEDD9 genomic region. Black boxes correspond to called binding events obtained using both MACS and SWEMBL algorithms. Full size image ChIP-qPCR analysis within the NEDD9 genomic locus (chr6:11,207,244–11,686,543) in MDA-MB-231 M1 showed strong TGFβ-induced binding of Smad2/3, SRF, MRTF-A and MRTF-B to intronic (R1 and R2) regions, and weak binding to the region 1 kb upstream of the short NEDD9 transcript (R3) ( Fig. 5d,e ). Under similar experimental conditions, we were unable to detect Smad2/3 or SRF binding to the NEDD9 locus in HCC1954 (data not shown). These data were confirmed by ChIP-sequencing in M1 MDA-MB-231 using a Smad2/3 antibody ( Fig. 5f ). These results show that in claudin low breast cancer cell lines TGFβ-mediated regulation of NEDD9 is achieved by Smad and MRTF-SRF binding within regulatory regions. NEDD9 mediates TGFβ-increased BTIC numbers We next asked whether NEDD9 is required to mediate an expansion of BTICs. To test this, we first generated MDA-MB-231 constitutively expressing a short-hairpin RNA targeting NEDD9 (MDA-MB-231-shNEDD9) ( Fig. 6a ). MS-ICs and LDA assays showed TGFβ-mediated increases in both self-renewal activity and BTIC numbers were significantly lower in MDA-MB-231-shNEDD9 clones compared with control cells ( Fig. 6b,c and Table 1 ). Moreover, forced overexpression of NEDD9 in HCC1954 increased the number of MS-ICs by approximately twofold compared with vector control-treated cells, suggesting that an increase in NEDD9 levels is sufficient to increase BTIC numbers ( Fig. 6d ). 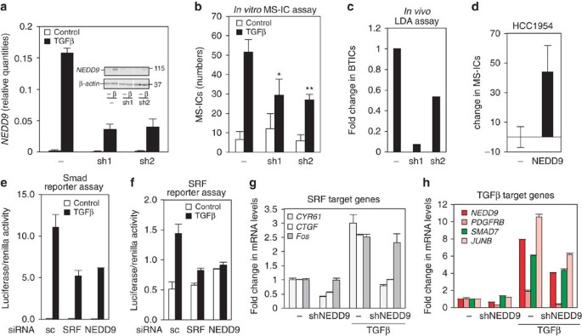Figure 6: TGFβ-induced expansion of the BTIC pool requires NEDD9. (a) qRT–PCR and western blot (insert) of NEDD9 in MDA-MB-231 transduced with empty vector control (−), or sh-NEDD9 (sh1 and sh2). NEDD9 expression was normalized against beta-2-microglobulin and expressed as arbitrary units. Error bars represent ±s.d. of three independent experiments. (b) Bar chart shows number of MS-ICs in M1 cultures of MDA-MB-231 clones described in (a). Error bars represent ±s.d. of at least three independent experiments. **TGFβ-treated empty vector (−) cultures versus TGFβ-treated sh-NEDD9 cultures,P<0.01. *TGFβ-treated empty vector (−) cultures versus TGFβ-treated sh-NEDD9 cultures,P<0.05 05 (Student'st-test). (c) Bars represent TGFβ-induced fold change in total number of TICs in M1 cultures of MDA-MB-231-clones described in (a) as compared with untreated empty vector M1 cultures (−) (see Table 1). (d) A NEDD9 expression vector was transiently transduced into HCC1954 cells. Results show percentage of change in MS-IC numbers in NEDD9 overexpressing HCC1954 M1 mammospheres (NEDD9) compared with control transduced cells (−). Error bars represent ±s.d. of independent experiments. (e) MDA-MB-231 cells were transfected in attached conditions with the indicated siRNAs and the TGFβ/Smad reporter vector (CAGA12-Luc). At 24 h post transfection, cells were passaged into a mammosphere culture and left untreated or treated with TGFβ (2.5 ng ml−1) for further 20 h. Luciferase activity was normalized to pGL-SV40 renilla transfection control. Error bars represent ±s.d. of three independent experiments. (f) MDA-MB-231 cells were transfected in attached conditions with the indicated siRNAs and the SRF reporter (p3DA.luc) and then treated as depicted in (d). Bar chart shows luciferase activity relative to renilla. Error bars represent ±s.d. of three independent experiments. (g) qRT–PCR of downstream target genes of SRF and (h) TGFβ/Smad signalling pathways in M1 MDA-MB-231 transduced with empty vector control (−) or sh-NEDD9 (shNEDD9) left untreated or treated with TGFβ (2.5 ng ml−1) for 1 h. Expression of mRNAs was normalized against beta-2-microglobulin and expressed as arbitrary units. Bars represent fold change in mRNA levels as compared with untreated empty vector transduced cells. Error bars represent ±s.d. of three independent experiments. Figure 6: TGFβ-induced expansion of the BTIC pool requires NEDD9. ( a ) qRT–PCR and western blot (insert) of NEDD9 in MDA-MB-231 transduced with empty vector control (−), or sh-NEDD9 (sh1 and sh2). NEDD9 expression was normalized against beta-2-microglobulin and expressed as arbitrary units. Error bars represent ±s.d. of three independent experiments. ( b ) Bar chart shows number of MS-ICs in M1 cultures of MDA-MB-231 clones described in ( a ). Error bars represent ±s.d. of at least three independent experiments. **TGFβ-treated empty vector (−) cultures versus TGFβ-treated sh-NEDD9 cultures, P <0.01. *TGFβ-treated empty vector (−) cultures versus TGFβ-treated sh-NEDD9 cultures, P <0.05 05 (Student's t -test). ( c ) Bars represent TGFβ-induced fold change in total number of TICs in M1 cultures of MDA-MB-231-clones described in ( a ) as compared with untreated empty vector M1 cultures (−) (see Table 1). ( d ) A NEDD9 expression vector was transiently transduced into HCC1954 cells. Results show percentage of change in MS-IC numbers in NEDD9 overexpressing HCC1954 M1 mammospheres (NEDD9) compared with control transduced cells (−). Error bars represent ±s.d. of independent experiments. ( e ) MDA-MB-231 cells were transfected in attached conditions with the indicated siRNAs and the TGFβ/Smad reporter vector (CAGA12-Luc). At 24 h post transfection, cells were passaged into a mammosphere culture and left untreated or treated with TGFβ (2.5 ng ml −1 ) for further 20 h. Luciferase activity was normalized to pGL-SV40 renilla transfection control. Error bars represent ±s.d. of three independent experiments. ( f ) MDA-MB-231 cells were transfected in attached conditions with the indicated siRNAs and the SRF reporter (p3DA.luc) and then treated as depicted in ( d ). Bar chart shows luciferase activity relative to renilla. Error bars represent ±s.d. of three independent experiments. ( g ) qRT–PCR of downstream target genes of SRF and ( h ) TGFβ/Smad signalling pathways in M1 MDA-MB-231 transduced with empty vector control (−) or sh-NEDD9 (shNEDD9) left untreated or treated with TGFβ (2.5 ng ml −1 ) for 1 h. Expression of mRNAs was normalized against beta-2-microglobulin and expressed as arbitrary units. Bars represent fold change in mRNA levels as compared with untreated empty vector transduced cells. Error bars represent ±s.d. of three independent experiments. Full size image NEDD9 coordinates a positive feedback loop in claudin low cells We hypothesized NEDD9 could, through its adaptor properties, be acting as a molecular scaffold to integrate TGFβ/Smad and MRTF-SRF signalling. Indeed, downregulation of NEDD9 blocks TGFβ-mediated increase in Smad and SRF transcriptional activity ( Fig. 6e,f ). Moreover, SRF transcriptional activation of two of the three tested MRTF-SRF targets ( CTGF and CYR61) was disrupted in sh-NEDD9-MDA-MB-231 mammosphere cultures at baseline and after TGFβ treatment ( Fig. 6g ). Similarly, the levels of several TGFβ/Smad-specific downstream targets were diminished in sh-NEDD9-MDA-MB-231 compared with vector control cells in the presence of TGFβ ( Fig. 6h ). These results suggest that a positive feedback autoregulatory loop involving TGFβ-mediated regulation of NEDD9 enables both TGFβ/Smad and MRTF-SRF pathway activity to converge at specific regulatory regions, including those within the NEDD9 genomic locus, to control the expression of a gene set involved in increasing BTIC numbers ( Supplementary Fig. S6 ). The results presented here represent a significant advance of our understanding of the dual role of the TGFβ pathway in regulating the growth and self-renewal of different subsets of normal and malignant mammary epithelial cells. We have identified a molecular mechanism where the NEDD9-Smad-SRF-dependent pathway regulates a TGFβ-specific transcriptional program (TβSC-A) associated with human stem cell features, which is necessary for TGFβ-induced BTIC activity. Previous observations showed TGFβ signalling has discordant effects on metastasis in mouse models [41] , [42] , [43] . Later, gene signatures specific of both active and inactive TGFβ pathway were correlated with poor outcome in breast cancer patients [44] , [45] . We have reconciled these apparently conflicting results by characterizing TGFβ pathway response signatures in cancer stem cell-enriched cultures. We identified two independent signatures (TβSC-A and TβSC-B) associated with TGFβ-mediated increase and decrease in BTIC activity, respectively, and then tested these signatures in human breast tumours looking for associations with clinical outcome. We observed that only TβSC-A is associated with a worse clinical outcome (and with stem cell features), showing that TGFβ prognostic signatures in breast cancer are ER-status independent, contrary to what was previously suggested [44] , but rather, associated with promotion of stem cell like features. We show claudin low breast cancer cells are more likely than other breast cancer subtypes to respond to TGFβ treatment by increasing BTIC numbers, hence, we investigated TGFβ effects in different human normal mammary cell subpopulations, which are presumed to give rise to different breast cancer subtypes [11] , [46] . TGFβ signalling in the mammosphere-forming and migratory capacity of human normal mammary epithelial CD49f + EpCAM neg/low cells (where MaSCs reside) has been recently reported [21] . Our data expands these in vitro observations by using a more robust in vivo experimental approach [30] , [31] . We show a short ( ex vivo) exposure to TGFβ increases in vivo MaSC/basal progenitor numbers independently of its cytostatic effects in the CD49f + EpCAM neg/low compartment and decreases the clonogenic capacity of luminal-restricted progenitors within the CD49f + EpCAM + compartment. These results show conservation between TGFβ effects in breast cancer and normal cell subtypes. TGFβ is a well-characterized EMT-inducing factor [47] . Because normal and malignant mammary stem cells show features of EMT and cells that have undergone EMT show properties of stem cells, the accepted model is that EMT and stemness are interlinked phenotypes [21] , [22] , [48] . Our observations show that TGFβ effects in BTIC are separable from EMT, as we observed TGFβ decreased BTIC activity in a basal-like cell line, and also mediated the induction of both EMT and an increase in the percentage of cells with a CD44 + /CD24 − phenotype. These results suggest mechanisms involved in TGFβ-induced changes on BTIC numbers are separable from those involved in promoting EMT and the CD44 + /CD24 − phenotype. We found active SRF is required for TGFβ-mediated regulation of TβSC-A genes. Two main families of SRF co-factors have been characterized: members of the ternary complex factor family activated by mitogen-activated protein kinase phosphorylation and members of the MRTF cofactors regulated by Rho-actin-dependent signals [49] . We focused on the Rho-actin-MRTF pathway for several reasons including that Smads had previously been shown to interact with MRTFs [50] , the Rho activity is induced by TGFβ in the claudin low MDA-MB-231 cell line but not in the basal HCC1954 cell line and also because others had shown in MDA-MB-231s SRF activity is regulated by Rho-actin-MRTF signals [40] . We dissected this pathway with the use of actin-modifiers, small-molecule inhibitors and siRNA technology and demonstrated that TGFβ-mediated effects on BTICs are dependent on Rho-actin-MRTF-SRF signalling. A functional cross-talk between the TGFβ pathway and NEDD9 had been previously described [17] , [51] , [52] , [53] . NEDD9 is also known to be an MRTF target and to regulate a member of the Rho-family of GTPases through the Rac guanine nucleotide exchange factor DOCK3 (refs 40 , 54 ). This suggests the existence of a functional cross-talk between NEDD9 and the Rho-actin-MRTF-SRF pathway as well. Here we show the ability of TGFβ to induce NEDD9 is both Smad and actin-MRTF-SRF-dependent, only in claudin low cancer cells. Moreover, we observe NEDD9 is required for TGFβ-induced Smad and SRF activity. Altogether, this data leads us to hypothesize that NEDD9, through a positive feedback loop, acts as a scaffold enabling the appropriate molecular interactions to connect TGFβ/Smad and Rho-actin-MRTF-SRF signals to coordinate the expression of genes involved in the expansion of the BTICs ( Supplementary Fig. S6 ). We observed NEDD9 was exclusively expressed in the human and mouse basal progenitor/MaSC populations, suggesting that the NEDD9 autoregulatory loop is also active in normal epithelial subpopulations and mediates TGFβ-dependent increase in epithelial stem cell numbers. Interestingly in MDA-MB-231, a claudin low cell line, MRTF-SRF transcriptional activation of several target genes was previously shown to be required for experimental metastasis [40] . Our data now reveals their transcriptional regulation by SRF is important in the maintenance of BTICs. Therefore, we propose that therapeutic targeting of both Rho family GTPases and TGFβ signalling might be an attractive strategy to eliminate breast cancer metastasis in claudin low breast cancers, by both suppressing the spreading of cancer cells and the self-renewal of the BTIC population. M1 mammosphere cultures Cells were processed to single-cell suspension from adherent cultures by trypsinization and cells were subsequently washed twice with PBS. A further wash in supplemented MEBM media was followed by filtration through a 40-μm cell strainer. Single cells were plated on ultra-low attachment plates (Corning) at a density of 50,000 cells ml −1 in supplemented MEBM media and grown for 7 days untreated or treated as indicated. M1 mammospheres were processed to single-cell suspension by trypsinization followed by neutralization using soyabean trypsin inhibitor 50 μg ml −1 (Roche). Cells were washed in PBS and resuspended in the same volume of supplemented MEBM as the initial primary mammosphere culture in the absence of treatment. MS-IC and CFC Assays For the MS-IC assay, the same number of single cells from the indicated cell lines were grown as M1 mammospheres for 7 days and left untreated or treated with single dose of TGFβ (2.5 ng ml −1 ) and/or of SB (10 μM) as indicated. Next, all single cells from these M1 cultures were grown in the absence of treatment as M2 mammospheres and total number of spheres counted 7–10 days later. CFC assay: same number of single cells from the indicated cell lines were grown as M1 mammospheres untreated or treated with TGFβ (2.5 ng ml −1 ) and/or of SB (10 μM) for 7 days as indicated. Aliquots of 100 μl from processed M1 cultures were plated onto collagen-coated plates (Iwaki cell biology) in 4 ml of CFC media (DMEM:F12 medium (Invitrogen) with 5% fetal bovine serum, 5 μg ml −1 insulin (Sigma) and 20 μg ml −1 of human recombinant epidermal growth factor (Invitrogen)). Colony growth was monitored, and plates fixed and stained with acetone/methanol (1:1) and Giemsa once colonies reached sufficient size to be counted with the naked eye. For the Limiting Dilution Assay, s ingle cells from processed M1 cultures were encapsulated in 20 μl gels; 7.8 parts 5:1 rat tail collagen:matrigel (Becton Dickinson), 2 parts 5×DMEM (Invitrogen) 0.2 parts 1 M NaOH (Sigma). Gels containing specific cell numbers were implanted under general anaesthesia into the inguinal mammary glands of NOD/SCID Il2rg −/− (NSG) mice. Tumour growth was monitored by luciferase imaging on the IVIS imaging system (Caliper life sciences) and manual palpation. Chromatin Immunoprecipitation Single-cell suspensions of volume 125 ml at a density of 1×10 5 cells per ml were incubated with stirring in disposable spinner flasks (Corning) for 4 days at 37 °C. Cell suspensions were treated with TGFβ for 1 h at 37 °C, where indicated, and ChIP was performed following the method outlined in Schmidt et al . [55] , using SRF rabbit polyclonal antibody (Santa Cruz Biotechnology Inc. sc-335 X) and smad2/3 rabbit polyclonal antibody (Santa Cruz Biotechnology Inc. sc-8332 X) and Protein G Dynabeads (Dynal). Dissociation and cell separation of human mammary tissue The use of human material followed protocols approved by the Research Ethics Committee. We collected tissue from women undergoing reduction mammoplasty surgery with informed consent and processed the tissue as previously described [56] . Cell sorting was performed as previously described with some minor modifications [56] . Briefly, we preblocked mammary cell suspensions in 1 ml of cold HF (Hanks (+Mg +Ca) + 2% Hepes + 2% fetal bovine serum) supplemented with 10% normal rat serum, and then labelled them with an allophycocyanin-conjugated rat antibody to human CD49f (clone GOH3, R&D Systems) and PE-conjugated antibody to human EpCAM PE (clone 9C4, Biolegend). We also labelled hematopoietic and endothelial cells with biotin-conjugated mouse antibodies to human CD45 (clone HI30, Biolegend) and human CD31 (clone WM59, eBiosciences), respectively, followed by R-phycoerythrin-conjugated streptavidin (BD Biosciences). We added propidium iodide (Sigma) at 1 mg ml −1 for live/dead cell discrimination. We performed all sorts on the FACS aria SORP (Becton Dickinson). Dissociation and cell separation of mouse mammary tissue Mammary glands from 8- to 14-week-old virgin female FVB mice were digested for 8 h at 37 °C in DMEM/F12 (Gibco: with L -glut and Hepes) with 300 U ml −1 collagenase and 100 U ml −1 hyaluronidase (Sigma). After vortexing and lysis of the red blood cells in NH 4 Cl, a single-cell suspension was obtained by sequential dissociation of the fragments by gentle pipetting for 1–2 min in 0.25% trypsin, and then 2 min in 5 mg ml −1 dispase II plus 0.1 mg ml −1 DNase I (Sigma). Cell separation was performed as previously described [32] . Briefly, cells were incubated for 10 min at 4 °C in 10% rat serum and stained with CD45-biotin (clone 30-F11 eBioscience), CD31-biotin (clone 390 eBioscience), Ter119-biotin (Ter119 eBioscience), BP-1-biotin, (Pharmingen), CD49f-AF488 (clone GoH3 Biolegend) and EpCAM-AF647 (clone G8.8 Biolegend). Cell death was determined by DAPI staining. Analysis of claudin low score in cell lines and tumour samples We used the cell line expression data from Neve et al . [57] and the nine-cell line claudin low signature from Prat et al . [9] to obtain a claudin low centroid and an ′others′ centroid, following the methodology in that paper [9] , [57] . Then, we normalized Illumina microarray data from the 11 cell lines analysed by us using beadarray [58] and annotated the probes using the latest files available in the re-annotation pipeline from Barbosa-Morais et al [59] , finding 741 of their signature genes in our arrays. With those genes, we computed the Spearman correlation of our cell lines to each of the centroids. The Claudin low score is the difference of the Spearman correlation value of our cell line expression data with the claudin low centroid and the Spearman correlation with the 'others' centroid (positive values indicate more Spearman correlation with the claudin low centroid and negative values more Spearman correlation with the 'others' centroid). We used Spearman correlation instead of Euclidean distance, as Prat et al . [9] did, because it is a more robust measure when dealing with expression levels of different microarray platforms. We employed the same methodology on the claudin low tumour predictor of Prat et al . [9] to classify the Metabric set of 997 breast tumours [36] , with 104 tumours classified as claudin low . Gene set enrichment analysis We ran GSEA v 2.07. [34] on our Metabric data set to test if TβSC-A signature is enriched in the claudin low tumours. As GSEA does not support gene sets that have both up- and downregulated genes, we used the subset of overexpressed genes in TβSC-A. For genes spanning several probes, we selected the best-annotated probe or the one showing more variability. The number of signature genes present in the Metabric microarray was 43. Regulatory network analysis ECRbase was used as the resource for TF-binding site annotation (see Supplementary Information ). We selected the subset of annotated TF-binding site that are conserved in human-opossum ECRs in the 5 Kb immediately upstream of the transcription start site. Thus, binding profiles for each position weight matrix (PWM) over all human ENSEMBL genes was constructed with a '1' indicating presence of motif in 5 Kb promoter region upstream of the gene, '0' otherwise. ENSEMBL IDs were mapped to Entrez Gene Ids. Next, for each TGFβ versus SB comparison, we extracted the regularized t -statistics of differential expression. Probes were mapped to Entrez Gene Ids and the t -statistics regressed against the binding profile of a PWM in a linear model [39] of the form t -statistics (TGFβ versus SB)=αB PWM + , from which a P -value of significance was derived. PWMs were then ranked according to significance of these P -values. Histogram of P -values showed skews towards small P -values suggesting significant differential activity of PWMs in response to TGFβ treatment. Plurinet analysis Genes from the plurinet network [35] were mapped to the Illumina array using Entrez ID identifiers and fold-change (FC) values (TGFβ versus SB) were extracted for each cell line. Next, we selected those that showed at least 1.25 FCs in either the two TβSC-A or TβSC-B cell lines, and only considered those where the direction of the FC was consistent between the two cell lines. The relaxation of the threshold to ±1.25 was justified based on the observation that the 'Plurinet' itself was derived from an algorithm that only demanded consistent directional changes over a local protein–protein interaction subnetwork without requiring the individual changes to be significant. Thus, for each set of cell lines, we could count the number of 'Plurinet' genes showing increases and decreases in TGFβ versus SB conditions. Any trend towards up- or downregulation of 'Plurinet' genes in the cell lines with TGFβ-induced BCSC activity against the other two cell lines could then be evaluated using a Fisher's exact test. Accesion codes: Microarray data have been deposited in ArrayExpress under the accession codes E-MTAB-516 and E-MTAB-1190 . How to cite this article: Bruna, A. et al . TGFβ induces the formation of tumour-initiating cells in claudin low breast cancer. Nat. Commun. 3:1055 doi: 10.1038/ncomms2039 (2012).